Variation at 3p24.1 and 6q23.3 influences the risk of Hodgkin’s lymphoma In addition to HLA, recent genome-wide association studies (GWASs) of Hodgkin’s lymphoma (HL) have identified susceptibility loci for HL at 2p16.1, 8q24.21 and 10p14. In this study, we perform a GWAS meta-analysis with published GWAS (totalling 1,465 cases and 6,417 controls of European background), and follow-up the most significant association signals in 2,024 cases and 1,853 controls. A combined analysis identifies new HL susceptibility loci mapping to 3p24.1 (rs3806624; P =1.14 × 10 −12 , odds ratio (OR)=1.26) and 6q23.3 (rs7745098; P =3.42 × 10 −9 , OR=1.21). rs3806624 localizes 5′ to the EOMES (eomesodermin) gene within a p53 response element affecting p53 binding. rs7745098 maps intergenic to HBS1L and MYB , a region previously associated with haematopoiesis. These findings provide further insight into the genetic and biological basis of inherited susceptibility to HL. Hodgkin’s lymphoma (HL) is a common lymph node cancer of germinal centre B-cell origin, which is characterized by malignant Hodgkin and Reed–Sternberg (HRS) cells mixed with a dominant background population of reactive lymphocytes and other inflammatory cells [1] . Although Epstein–Barr virus (EBV) infection may be causally related to a number of cases, there is little evidence to support the involvement of other environmental risk factors [2] . Evidence for inherited genetic influence on susceptibility is provided by the increased familial risk and very high concordance between monozygotic twins [3] . Although the risk of HL is well recognized to be influenced by HLA genotype variation within the major histocompatibility complex, much of the familial risk is thought to be the consequence of non-HLA genotype variation. Support for this hypothesis has come from recent genome-wide association studies (GWASs) of HL that, in addition to demonstrating multiple HLA associations [4] , [5] , [6] , [7] , have identified non-HLA susceptibility loci at 2p16.1 ( REL ), 8q24.21 and 10p14 ( GATA3 ) [7] . In this study to identify additional susceptibility loci for HL, we conducted an independent primary scan of German patients with classical HL (cHL) and performed a genome-wide meta-analysis with one previously published GWAS of UK cHL patients. The most significant single nucleotide polymorphisms (SNPs) were analysed in two additional series totaling 2,024 cases and 1,853 controls. A combined analysis identified new HL susceptibility loci mapping to 3p24.1 and 6q23.3. GWAS and meta-analysis In the primary scan (German-GWAS), 1,001 cHL cases, ascertained by the German Hodgkin Study Group during 1998–2007, were genotyped using the Illumina Human OmniExpress-12 v1.0 arrays. For controls, we used genotype data on 1,226 individuals enrolled into the Heinz Nixdorf Recall study genotyped using Illumina OmniExpress-12 v1.0. A total of 133 case samples were removed during quality control steps for reasons including a failure to genotype, duplicates, closely related individuals or non-CEU ancestry (CEU-Utah residents with Northern and Western European ancestry; Figs 1 and 2 ). 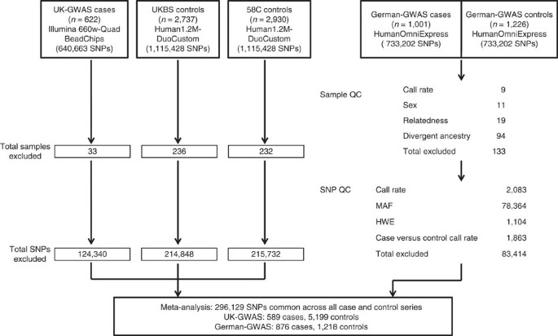Figure 1: GWAS data quality control. Details are provided of the samples and SNPs used in UK-GWAS and quality control of German-GWAS. Quality control of UK-GWAS reported in previously published work42. Figure 1: GWAS data quality control. Details are provided of the samples and SNPs used in UK-GWAS and quality control of German-GWAS. Quality control of UK-GWAS reported in previously published work [42] . 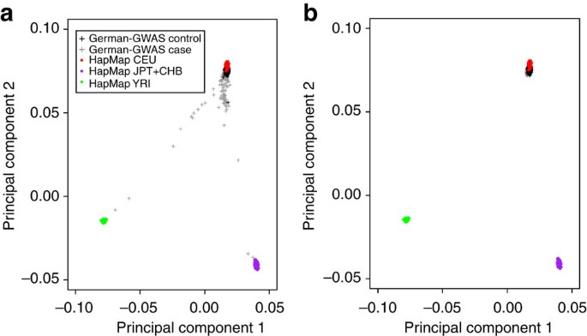Figure 2: Identification of samples of non-European origin for the German GWAS. The first two principal components of the analysis are plotted in each figure. (a) German controls (black crosses) and cases (grey crosses) are shown together with the HapMap CEU (Utah residents with Northern and Western European ancestry) individuals (red), CHB (Han Chinese in Beijing)+JPT (Japanese in Tokyo) individuals (purple) and YRI (Yoruba in Ibadan) individuals (green). (b) The same plot is shown after the removal of cases and controls of non-European origin. Respective data on UK-GWAS provided in previously published work42. Full size image Figure 2: Identification of samples of non-European origin for the German GWAS. The first two principal components of the analysis are plotted in each figure. ( a ) German controls (black crosses) and cases (grey crosses) are shown together with the HapMap CEU (Utah residents with Northern and Western European ancestry) individuals (red), CHB (Han Chinese in Beijing)+JPT (Japanese in Tokyo) individuals (purple) and YRI (Yoruba in Ibadan) individuals (green). ( b ) The same plot is shown after the removal of cases and controls of non-European origin. Respective data on UK-GWAS provided in previously published work [42] . Full size image The UK-GWAS has been previously reported [7] ; briefly, 622 cHL cases were genotyped using Illumina 660w-Quad BeadChips. Genotype frequencies were compared with publicly accessible genotype data generated by the UK Wellcome Trust Case–Control Consortium 2 study of 2,930 individuals from the 1958 British Birth Cohort (58C) and 2,737 individuals from the UK Blood Service collections that had been genotyped using the Illumina Human1.2M-Duo Custom_v1 Array. There was no evidence of systematic bias between these two series, which were combined to provide genotype data for 5,667 controls [7] . Quality control steps for the UK GWAS have been previously reported [7] . After filtering of genotype data from each GWAS on the basis of pre-specified quality control measures, 296,129 autosomal SNPs were common to both case–control series. Quantile–quantile plots of the genome-wide Armitage trend test χ 2 -values showed that there was minimal inflation of the test statistics rendering substantial cryptic population substructure or differential genotype calling between cases and controls unlikely in either GWAS (genomic control inflation factor [8] , λ gc =1.03 and 1.09 in UK and German-GWAS, respectively; Fig. 3 ). In the combined analysis under a fixed effects model, we identified 27 SNPs in 21 genomic regions not previously associated with cHL risk, which showed good evidence for a relationship (that is, P <5.0 × 10 −5 fixed effects model inverse-variance weighted meta-analysis test; Fig. 4 , Supplementary Table S1 ). 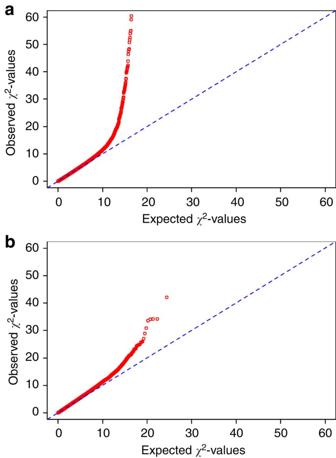Figure 3: Quantile–quantile (Q–Q) plots ofχ2-values for association. (a) UK cases and UK controls (λ=1.03); (b) German cases and German controls (λ=1.09). Figure 3: Quantile–quantile (Q–Q) plots of χ 2 -values for association. ( a ) UK cases and UK controls ( λ =1.03); ( b ) German cases and German controls ( λ =1.09). 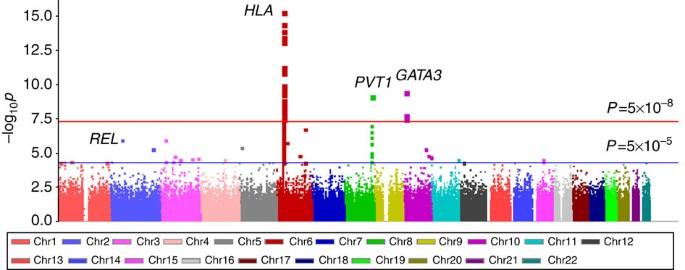Figure 4: Genome-wideP-values plotted against their respective chromosomal positions. Shown are the genome-wideP-values (two-sided) obtained using the Cochran–Armitage trend test from 296,129 autosomal SNPs in 1,465 HL cases and 6,417 controls. The red horizontal line represents the genome-wide significance threshold level (P=5.0 × 10−8). The blue horizontal line represents the significance threshold at which SNPs were selected for genotyping in UK-replication 1 (P<5.0 × 10−5). Previously identified risk loci atREL, HLA, PVT1andGATA3are labelled. Full size image Figure 4: Genome-wide P -values plotted against their respective chromosomal positions. Shown are the genome-wide P -values (two-sided) obtained using the Cochran–Armitage trend test from 296,129 autosomal SNPs in 1,465 HL cases and 6,417 controls. The red horizontal line represents the genome-wide significance threshold level ( P =5.0 × 10 −8 ). The blue horizontal line represents the significance threshold at which SNPs were selected for genotyping in UK-replication 1 ( P <5.0 × 10 −5 ). Previously identified risk loci at REL, HLA, PVT1 and GATA3 are labelled. Full size image Replication genotyping To validate these findings, we genotyped the SNP showing the best evidence of association in each of the 21 regions in the UK-replication 1 series. In the combined analysis, rs3806624 and rs7745098 showed consistent evidence for an association with HL risk applying a fixed effects model to Armitage trend test statistics (combined P -value<5.0 × 10 −7 ; Supplementary Table S2 ) and these SNPs were genotyped in the UK-replication 2 series. In a combined analysis of all data sets, the rs3806624 and rs7745098 associations were statistically significant on a genome-wide basis (that is, P <5.0 × 10 −8 fixed effects model inverse-variance weighted meta-analysis test; Fig. 5 ; Supplementary Table S3 ). 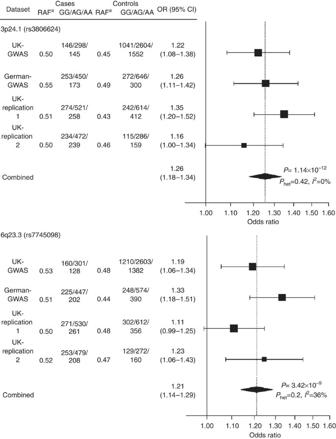Figure 5: Plot of the ORs of HL associated with rs3806624 and rs7745098. Studies were weighted according to the inverse of the variance of the log of the OR calculated by unconditional logistic regression. Horizontal lines: 95% confidence intervals (95% CI). Box: OR point estimate; its area is proportional to the weight of the study. Diamond (and broken line): overall summary estimate under fixed effects model, with CI given by its width. Unbroken vertical line: null value (OR=1.0). Figure 5: Plot of the ORs of HL associated with rs3806624 and rs7745098. Studies were weighted according to the inverse of the variance of the log of the OR calculated by unconditional logistic regression. Horizontal lines: 95% confidence intervals (95% CI). Box: OR point estimate; its area is proportional to the weight of the study. Diamond (and broken line): overall summary estimate under fixed effects model, with CI given by its width. Unbroken vertical line: null value (OR=1.0). Full size image rs3806624 localizes to 3p24.1 (27,764,623 bp; combined P =1.14 × 10 −12 fixed effects model inverse-variance weighted meta-analysis test, odds ratio (OR)=1.26) 5′ to the EOMES (eomesodermin; MIM:604615) gene ( Fig. 6 ) within a 110-kb region of linkage disequilibrium (LD). rs7745098 localizes to 6q23.3 (135,415,004 bp; combined P =3.42 × 10 −9 fixed effects model inverse-variance weighted meta-analysis test; OR=1.21) and maps intergenic to HBS1L (HBS1-like protein; MIM 612450) and MYB (V-MYB avian myeloblastosis viral oncogene homologue; MIM:189990) genes. To explore the 3p24.1 and 6q23.3 regions of association further, we imputed unobserved genotypes in GWAS cases and controls using 1,000 genomes data. This analysis did not reveal a significantly stronger association at 3p24.1 and 6q23.3 to that provided by rs3806624 and rs7745098, respectively ( Fig. 6 ). 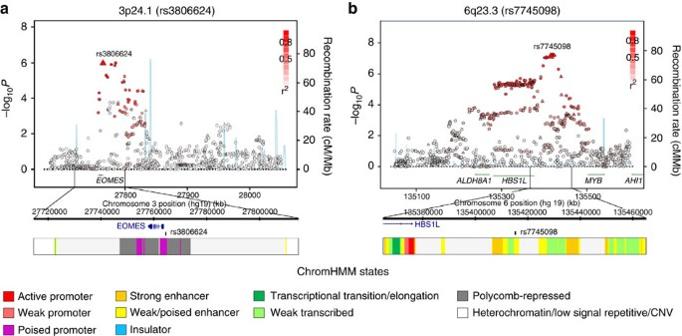Figure 6: Regional plots of 3p24.1 and 6q23.3 associations with recombination rates and chromatin state segmentation tracks. (a) 3p24.1 and (b) 6q23.3. Association results of both genotyped (triangles) and imputed (circles) SNPs in the GWAS samples and recombination rates for rates. −log10P=values (yaxis) of the SNPs are shown according to their chromosomal positions (xaxis). The top genotyped SNP in each combined analysis is shown as a large triangle and is labelled by its rsID. Colour intensity of each symbol reflects the extent of LD with the top genotyped SNP; white (r2=0) through to dark red (r2=1.0) Genetic recombination rates, estimated using HapMap Utah residents of Western and Northern European ancestry (CEU) samples, are shown with a light blue line. Physical positions are based on NCBI Build 37 of the human genome. Also shown are the relative positions of genes and transcripts mapping to the region of association. Genes have been redrawn to show the relative positions; therefore, maps are not to physical scale. The lower panel shows the exons and introns of the gene of interest; observed SNP and chromatin state segmentation track (ChromHMM). Figure 6: Regional plots of 3p24.1 and 6q23.3 associations with recombination rates and chromatin state segmentation tracks. ( a ) 3p24.1 and ( b ) 6q23.3. Association results of both genotyped (triangles) and imputed (circles) SNPs in the GWAS samples and recombination rates for rates. −log 10 P =values ( y axis) of the SNPs are shown according to their chromosomal positions ( x axis). The top genotyped SNP in each combined analysis is shown as a large triangle and is labelled by its rsID. Colour intensity of each symbol reflects the extent of LD with the top genotyped SNP; white ( r 2 =0) through to dark red ( r 2 =1.0) Genetic recombination rates, estimated using HapMap Utah residents of Western and Northern European ancestry (CEU) samples, are shown with a light blue line. Physical positions are based on NCBI Build 37 of the human genome. Also shown are the relative positions of genes and transcripts mapping to the region of association. Genes have been redrawn to show the relative positions; therefore, maps are not to physical scale. The lower panel shows the exons and introns of the gene of interest; observed SNP and chromatin state segmentation track (ChromHMM). Full size image Subtype analysis HL is biologically heterogeneous [2] , something reflected in the histology of tumour subtypes. In addition, a hallmark of cHL epidemiology is the bimodal age-specific incidence, and it has been argued that the disease in young adults and older adults are aetiologically different; in particular, there is a lower prevalence of EBV in young cHL cases (that is, <40 years), with ~70% of mixed cellularity cHL being EBV-positive compared with only ~20% of nodular sclerosis cHL. We assessed by case-only analysis the relationship between cHL and sex, age, histology and EBV status and rs3806624, rs7745098 genotype ( Supplementary Table S4 ). Using case-only logistic regression, a strong association was seen between rs3806624 and age at diagnosis of cHL with an increased prevalence of the G risk allele in cases diagnosed before age 40 ( P =8.35 × 10 −4 Wald test on the coefficient). None of the other associations were statistically significant. Impact of SNPs on heritability of HL There was no evidence of significant interaction between either rs3806624 or rs7745098 and the previously identified risk loci at 2p16.1 (rs1432295), 6p21.32 (rs6903608), 8q24.21 (rs2608053), 8q24.21 (rs2019960) and 10p14 (rs501764), an observation compatible with each locus having an independent effect on HL risk. To quantify the impact of the known loci on the heritability associated with common variation at the non-HLA-linked loci (3p24.1, 6q23.3, 2p16.1, 8q24.21, 8q24.21 and 10p14), using data from UK-GWAS and German-GWAS we computed the receiver operator characteristic associated with rs3806624, rs7745098, rs1432295, rs2608053, rs2019960 and rs501764 genotypes. The area under the curve corresponding to these variants was 0.63 translating into them collectively accounting for ~7% of the familial risk. Deciphering association signals The functional basis of many GWAS signals can be ascribed to sequence changes having an impact on gene expression and sequence conservation in non-coding regions has been shown to be a good predictor of cis -regulatory sequences. Using publicly accessible expression quantitative trait loci (eQTL) data on lymphoblastoid cell lines (LCLs) and T cells, we examined whether either rs3806624 or rs7745098 genotype is associated with differential expression. Although the associations identified did not show consistent statistically significant evidence of cis -acting regulatory effects in publicly accessible eQTL data, this does not preclude the possibility that the causal variants at these disease loci have subtle effects on expression, as the dynamic range of transcripts is small. Further, it is likely that only a cumulative long-term imbalance in expression of target genes will influence cHL development, and expression differences may be relevant only to a specific subpopulation of B cells, which may not be well modelled by EBV-transformed lymphocytes. To examine whether any directly typed or imputed SNPs lie within or very close to a putative transcription factor-binding/enhancer element, we conducted a bioinformatic search of each region of association. rs3806624 maps within a predicted promoter with histone marks of regulatory elements associated with promoters shown in multiple cell types; rs7745098 is within a highly evolutionary conserved region with predicted weak enhancer activity ( Fig. 6 ; Supplementary Table S5 ). We have identified common variants on chromosome 3p24.1 and 6q23.3 that influence the risk of cHL. Some (HLA; 8q24.21 rs2608053; 5q31 rs20541) but not all of the previously identified risk loci for cHL have differential effects according to histology and EBV status [5] , [7] . Our study findings suggest that 3p24.1 and 6q23.3 have generic effects on the development of cHL akin to 10p14 variation [7] . As rs3806624 localizes 5′ to the EOMES gene and there are no other known genes within this region of LD, there is a high likelihood that the functional basis of the 3p24.1 association is mediated through variation in this gene a priori. Although we cannot exclude the possibility that rs3806624 is simply acting as a marker for the 3p24.1 association, interrogation of the association signal through imputation failed to recover a statistically stronger association. Moreover, as rs3806624 maps within a p53 response element affecting p53 binding, with the risk allele G displaying weaker binding than the A allele [9] it is likely that the SNP is causal. EOMES is a member of the TBR1 subfamily of T-box genes that have a critical role in embryogenesis and pluripotency. Although EOMES seems important in extranodal natural killer/T-cell lymphoma [10] , evidence for a role of EOMES in cHL aetiology is currently lacking. A high proportion of the reactive infiltrate in cHL tumours is however composed of T helper 2 (Th2)-like cells with a T regulatory phenotype and crosstalk between these cells and the HRS cells seem essential for tumour growth [11] . Notably, a key characteristic of HRS cells is the production of cytokines and chemokines driven by GATA3 and T-bet expression and other T-cell transcription factors [12] . EOMES is necessary for full effector differentiation of CD8+ T cells complementing the actions of T-bet and acting as a key regulatory gene in the development of cell-mediated immunity [13] ; CD8+ T cells deficient in Eomes and T-bet fail to differentiate into functional killers required for viral defence [14] . Differential expression of Eomes and T-bet seem to facilitate the cooperative maintenance of the pool of antiviral CD8+ T cells during chronic viral infection [15] , something highly pertinent to cHL. CD44-positive memory Th2 cells expressing interleukin-5 (Il5) have lower levels of Eomes than Th2 cells lacking Il5 expression [16] . We have previously shown that variation at GATA3 is a determinant of cHL risk [7] . Downregulation of Eomes is required for Il5 expression and Eomes suppresses Gata3 transcriptional activity by inhibiting Gata3 binding to the Il5 promoter [16] . These findings support a role for an extended pathway involving GATA3 and EOMES genes in the aetiology of cHL. rs170934 that maps 314 kb telomeric to EOMES (28,079,085 bp) has previously been shown to be a risk factor for multiple sclerosis [17] . Intriguingly, familial clustering of HL and multiple sclerosis is seen suggesting a common aetiological basis to both diseases [18] . This coupled with the biology of EOMES strengthens the link between autoimmunity and HL and raises the possibility of a model by which T-cell activation has a role in both diseases through aberrant antigenic response. rs7745098 maps intergenic to HBS1L and MYB , a region of the genome, which has previously been reported to have a substantial role in haematopoiesis with polymorphisms influencing platelet [19] , white cell count [20] and haemoglobin levels [21] . Although evidence for a role for HBS1L in haematological malignancy is lacking, MYB, through its interaction with p300, controls the proliferation and differentiation of haematopoietic stem and progenitor cells. Although we do not find evidence of cis -acting regulatory effects in publicly accessible eQTL data from analysis of LCLs or T cells, steady-state levels of RNA in lymphocytes at a single time point and in cycling mature cells may not adequately capture the impact of differential expression in tumorigenesis. In summary, we have identified new risk loci at 3p24.1 and 6p22 for cHL, which provide additional insight into the development of this B-cell malignancy. Ethics Collection of samples and clinicopathological information from subjects was undertaken with informed consent and relevant ethical review board approval in accordance with the tenets of the Declaration of Helsinki (in the United Kingdom, the Royal Marsden Hospital NHS Trust and Multicentre Research Ethics Committee; in Germany, The Ethics committee of the University of Cologne). Discovery subjects The German-GWAS comprised 1,001 cHL cases (597 men; mean age at diagnosis=34.8 years, s.d.=12.3) ascertained by the German Hodgkin Study Group during 1998–2007. Cases were genotyped using Illumina Human OmniExpress-12 v1.0 arrays according to the manufacturer’s protocols (Illumina, San Diego, USA). For controls, we used genotype data on 1,226 individuals enrolled into the Heinz Nixdorf Recall study genotyped using Illumina OmniExpress-12 v1.0. The UK-GWAS has been previously reported [7] ; briefly, 622 cHL cases (63 men, mean age at diagnosis=24.4 years, s.d.=9.6) were genotyped using Illumina 660w-Quad BeadChips. Genotype frequencies were compared with publicly accessible genotype data generated by the UK Wellcome Trust Case–Control Consortium 2 (ref. 22 ) study of 2,930 individuals from the 1958 British Birth Cohort (58C) [23] and 2,737 individuals from the UK Blood Service collections that had been genotyped using the Illumina Human1.2M-Duo Custom_v1 Array. There was no evidence of systematic genotyping bias between these two series, which were combined to provide genotype data for 5,667 controls [7] . Quality control of GWAS data sets DNA samples with GenCall scores <0.25 at any locus were considered ‘no calls’. A SNP was deemed to have failed if <95% of DNA samples generated a genotype at the locus. A sample was deemed to have failed if <95% of SNPs were successfully genotyped. The same quality control metrics on the German-GWAS data were applied as in the UK-GWAS [7] . We computed identity-by-state (IBS) probabilities for all pairs (cases and controls) to search for duplicates and closely related individuals amongst samples (defined as IBS≥0.80, thereby excluding first-degree relatives). For all identical pairs the sample having the highest call rate was retained. To identify individuals who might have non-Western European ancestry, we merged our case and control data with phase II HapMap samples (60 Western European (CEU), 60 Nigerian (YRI), 90 Japanese (JPT) and 90 Han Chinese (CHB)). For each pair of individuals, we calculated genome-wide IBS distances on markers shared between HapMap and our SNP panel, and used these as dissimilarity measures on which to perform principal component analysis. We filtered out SNPs having a minor allele frequency <1% and a call rate <95% in cases or controls. We also excluded SNPs showing departure from Hardy–Weinberg equilibrium at P <1 × 10 −7 ( χ 2 -test with 1 degree of freedom or Fisher’s exact test if a cell count was <5). After stringent quality control filtering ( Fig. 1 ), we analysed 296,129 autosomal SNPs, common to all cases and controls, in 1,465 cHL cases and 6,417 controls. Cluster plots were manually inspected for all SNPs considered for replication. Replication series and genotyping UK-replication 1 comprised 1,071 UK patients diagnosed with cHL of either mixed cellularity HL (269 men; mean age at diagnosis 46.9 years, range 15–86) or nodular sclerosis HL (306 men; mean age at diagnosis 31.4 years, range 15–49). The patients were ascertained through the National Study of Hodgkin’s Lymphoma Genetics ( http://www.public.ukcrn.org.uk ), an ongoing study of HL established in 2008. Controls were healthy individuals recruited through the National Study of Colorectal Cancer Genetics ( n =1,186,367 men; mean age 58.6) [24] and the Royal Marsden Hospital Trust/Institute of Cancer Research Family History and DNA Registry ( n =102,17 men; mean age 59.3) with no personal history of malignancy. Both cases and controls were UK residents and had self-reported European ancestry. UK-replication 2 comprised 953 cHL cases (defined according to ICD10 C81.0-3; 290 men, mean age of diagnosis (AOD)=38 years, s.d.=16 years) ascertained from the Scotland and Newcastle Epidemiological Study of Hodgkin Disease (SNEHD), the Young Adult Hodgkin Case–Control Study (YHCCS) and the Epidemiology and Cancer Statistics Group Lymphoma Case–Control Study (ELCCS; http://www.elccs.info ). Full details of the SNEHD, YHCCS and ELCCS studies were provided previously. Briefly, SNEHD involved ascertainment of incident cases from Scotland and Northern England during 1993–1997. YHCCS was based on newly diagnosed cases aged 16–24 years from Northern England during 1991–1995. ELCCS comprised cases residing in the north of England aged 16–69 years, with newly diagnosed, non-human immunodeficiency virus-related HL, during 1998–2003. UK population controls were obtained from SNEHD, YHCCS and ELCCS ( n =565, 326 men, mean age 41 years, s.d.=17 years). The EBV status of cHL tumours was determined by immunohistochemical staining for EBV latent membrane antigen-1 and/or EBV EBV-encoded RNA in situ hybridization using sections of paraffin-embedded material. Genotyping was performed using competitive allele-specific PCR KASP chemistry (LGC, Hertfordshire, UK). Primers used are listed in Supplementary Table S6 . To ensure quality of genotyping in all assays, at least two negative controls and 6–7% duplicates (showing a concordance >99.9%) were genotyped. Call rates were >95% per 384-well plate for each SNP; cluster plots were visually examined by two researchers. Statistical and bioinformatic analysis Main analyses were undertaken using R (v2.10.1; http://www.r-project.org ), Stata v.10 (State College, Texas, USA) and PLINK (v1.07) [25] software. The association between each SNP and risk was assessed by the Cochran–Armitage trend test. The adequacy of the case–control matching and possibility of differential genotyping of cases and controls were formally evaluated using quantile–quantile plots of test statistics. The inflation factor λ was based on the 90% least significant SNPs [8] . ORs and associated 95% confidence intervals were calculated by unconditional logistic regression. Meta-analysis was conducted using standard methods under a fixed effects model [26] , [27] . Cochran’s Q statistic to test for heterogeneity and the I 2 statistic to quantify the proportion of the total variation because of heterogeneity were calculated [28] . I 2 -values≥75% are considered characteristic of large heterogeneity [28] . Associations by age, sex, histology and EBV status were examined by case-only analyses. Assuming a sibling relative risk of 3.93 (ref. 29 ) and a prevalence of 2.8 × 10 −5 (Surveillance Epidemiology and End Results data), we made use of receiver operator characteristic curve analysis [30] to estimate the proportion of the genetic variance on the liability scale attributable to variation at rs3806624, rs7745098, rs1432295, rs6903608, rs2608053, rs2019960 and rs501764. Prediction of untyped SNPs was carried out using IMPUTEv2 (ref. 31 ) based on the 1,000 genomes phase 1 integrated variant set (b37) from March 2012. Imputed data were analysed using SNPTEST v2 to account for uncertainties in SNP prediction [32] . LD metrics were calculated in PLINK (ref. 25 ) using 1,000 genomes data and plotted using SNAP [33] . LD blocks were defined on the basis of HapMap recombination rate (cM/Mb) as defined using the Oxford recombination hotspots [34] and on the basis of distribution of confidence intervals defined by Gabriel et al . [35] To explore the epigenetic profile of association signals, we made use of chromatin state segmentation in LCL data generated by the ENCODE Project [36] . The states were inferred from ENCODE Histone Modification data (H4K20me1, H3K9ac, H3K4me3, H3K4me2, H3K4me1, H3K36me3, H3K27me3, H3K27ac and CTCF) binarized using a multivariate Hidden Markov Model. We made use of RegulomeDB [37] and HaploReg [38] to examine whether any of the SNPs or their proxies (that is, r 2 >0.8 in 1,000 genomes CEU reference panel) annotate putative transcription factor-binding/enhancer elements. Relationship between SNP genotype and mRNA expression To examine for a relationship between SNP genotype and expression, we made use of publicly available expression data generated on LCLs and T cells from HapMap3, Geneva and the MuTHER pilot data using Sentrix Human-6 Expression BeadChips (Illumina) [39] , [40] , [41] . How to cite this article: Frampton, M. et al . Variation at 3p24.1 and 6q23.3 influences the risk of Hodgkin’s lymphoma. Nat. Commun. 4:2549 doi: 10.1038/ncomms3549 (2013).